Investigation of femtosecond collisional ionization rates in a solid-density aluminium plasma The rate at which atoms and ions within a plasma are further ionized by collisions with the free electrons is a fundamental parameter that dictates the dynamics of plasma systems at intermediate and high densities. While collision rates are well known experimentally in a few dilute systems, similar measurements for nonideal plasmas at densities approaching or exceeding those of solids remain elusive. Here we describe a spectroscopic method to study collision rates in solid-density aluminium plasmas created and diagnosed using the Linac Coherent light Source free-electron X-ray laser, tuned to specific interaction pathways around the absorption edges of ionic charge states. We estimate the rate of collisional ionization in solid-density aluminium plasmas at temperatures ~30 eV to be several times higher than that predicted by standard semiempirical models. A knowledge of the rate at which electrons are removed from, or recombine with, atoms and ions in a plasma is of fundamental importance in the understanding and prediction of plasma formation and dynamics. Changes in the charge state can occur via many processes, for example, interactions with photons, charge exchange, Auger decay and—of interest here—via collisional ionization with unbound electrons within the system. For weakly coupled systems, where the thermal energy of the charged components greatly exceeds their mean energy of coulomb interaction, the plasma can be treated as close to ‘ideal’, and it is commonly assumed when calculating collisional ionization rates that the collisions can be treated as binary, that is, that collective many-body effects play a negligible role in determining the dynamics of the interaction. Under such an assumption, cross-sections can be calculated via the binary scattering theory, and by integrating these over the electron density and temperature distribution, the appropriate collision rates can be obtained. For many configurations these rates can be calculated theoretically within the relativistic distorted-wave approximation framework, which yields accurate results for high-temperature, highly ionized plasmas. This method is currently implemented in the widely used HULLAC [1] and FAC [2] atomic codes, but can be further refined to a range of increasingly complex plasma conditions (see ref. 3 , and references therein). However, given the very large number of possible different ionization configurations, and/or the need for a comprehensive treatment of further effects, such as inner-shell excitation and autoionization, which can quickly become computationally cumbersome, empirical or semiempirical formulae, such as those in ref. 4 , 5 , 6 , 7 , are popular for use within collisional-radiative modelling codes (for example, FLYCHK [8] and SCFLY [9] , CRETIN [10] , CRModel [11] and ABAKO [12] ). Owing to the foundational link between rates and dynamics, collisional ionization cross-sections for isolated atoms and ions have been thoroughly investigated experimentally over the past half century using a variety of techniques such as the crossed-beam method [13] , or directly via plasma spectroscopy of well-defined low-density systems [14] , [15] . The rate of collisional ionization follows directly from the cross-section once the number and energy of the colliders are known, via the temperature-dependent electron distribution function. In contrast, our understanding of the rate of collisional ionization in dense, strongly coupled plasmas, where the binary-collision model breaks down, is woefully inadequate. Such plasmas are prevalent throughout the Universe within stellar environments—for example, the conditions half-way to the centre of the sun are equivalent in density to that of a typical solid, but with temperatures of order 100 eV. A number of theoretical approaches have been taken in an attempt to model collisions within such systems. Indeed, it is predicted that many-body effects such as plasma screening and ionization potential depression (IPD) can already have a significant effect on these rates at electron densities of 10 21 cm −3 (refs 16 , 17 ), increasing them several times over and above those that would be predicted by a more classical binary approach. As experiments using intense, short-pulse lasers to heat solid targets, as well as inertial confinement fusion investigations, routinely deal with nonequilibrium plasmas at even higher electron densities, in the range of 10 23 –10 25 cm −3 (refs 18 , 19 ), an understanding of how collisional ionization processes are affected in a dense plasma environment is of great practical importance [20] , [21] . While a considerable amount of theoretical work has been carried out on calculating collisional ionization rates in dense plasmas, there is a dearth of experimental data in this regime. In part, this is because of the difficulty of producing highly ionized, dense and hot plasmas under well-known conditions, but also because the measurement of collision rates cannot generally be isolated from other competing transitions and recombinations, such that a good understanding of all the processes in the plasma system is required to investigate any single one. Moreover, for most conditions of interest in dense plasmas far from equilibrium, Auger recombination, electron collisional ionization and other electronic processes occur on femtosecond timescales, severely limiting the feasibility of direct, time-resolved investigations. It is in the above context that we describe here an experimental method to investigate the collisional ionization rates under warm- and hot-dense plasma conditions with well-defined electron densities and temperatures. We show that the commonly used semiemprical models [4] , [5] , implemented in many plasma-kinetics codes, underestimate the rate of collisional ionization by a considerable margin—a trend predicted by the theoretical investigations cited above [16] , [17] , [21] . As we will describe, our method relies on heating a solid target with the Linac Coherent Light Source (LCLS) X-ray free-electron laser (FEL). We exploit the short duration of the X-ray pulse to ensure that the plasma we create and study is heated isochorically to well-defined conditions, and the tunability of the LCLS photon energy to allow us, via X-ray-driven emission spectroscopy, to investigate specific collisional ionization rates within the system. Experiment We use the LCLS FEL [22] to create a hot and dense Al plasma on ultrashort timescales using X-ray irradiation of 1-μm-thick foil targets at peak intensities reaching 10 17 W cm −2 . The X-ray wavelength is tuned over a range of values around the K-edges of the various ionization stages of Al, so that the predominant absorption pathway for the X-rays is K-shell photoionization, leading to the creation of a core hole in the 1 s state. This K-shell hole subsequently recombines within a few femtoseconds, mainly via Auger decay from the L-shell, so that the energy of the X-ray pulse is efficiently retained, and the system is rapidly heated to peak temperatures approaching 200 eV, at solid density, within the duration of the pulse. The experiment, and the properties of the plasma created, has been described in detail elsewhere [23] , [24] , [25] . The main experimental diagnostic is X-ray emission spectroscopy in the Al K α region of the spectrum in the range 1,460–1,600 eV, obtained via an ADP (101) crystal spectrometer with spectral resolution of ~1.3 eV. Since the system is driven to temperatures not high enough to thermally ionize the K-shell, the K α emission is driven solely by the X-ray beam, and the spectra carry information on the system exclusively within the duration of the X-ray pulse, which is of ~80 fs. Because of these short timescales, the ions do not have time to move more than a fraction of the lattice spacing, and the heating of the sample is isochoric with a well-known ion density throughout the entire time of emission. The electrons, on the other hand, equilibrate very quickly, and collisional ionization was observed to play an important role in their thermalization within the duration of the pulse [23] . The experimentally measured spectra for a range of X-ray irradiation photon energies are shown in Fig. 1 . The various emission lines correspond to different charge states of an Al ion containing one hole in the K-shell and an additional number of holes in the L-shell. The first line in Fig. 1 , denoted by IV, is emitted from a system containing initially a single K-shell hole and a fully filled L-shell. The three M-shell electrons are considered to be pressure-ionized in metallic Al. Since emission from line IV can only be observed if a 1 s electron is photoionized from an ion with charge state 3 + , the onset of this emission can be used to determine the K-shell ionization energy of the said charge state. Similarly, emission from V is determined by the K-edge of charge state 4 + , and so on, for all possible occupations of the L-shell. Therefore, by observing the intensity of an emission line as a function of the photon energy of the X-ray pump, the positions of the K-edges can be extracted from the data for a range of specific ionic charge states, a result that has recently led to the reporting of the first direct measurement of the IPD in a dense plasma [25] . 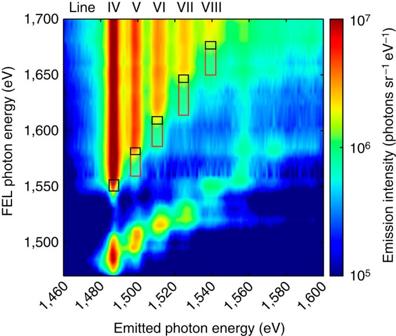Figure 1: Experimental emission spectra. Experimentally measured Kαintensities as a function of the spectrally resolved emission (horizontal axis) and X-ray pump photon energy (vertical axis)23,24. Emission from Al charge states 4+to 8+are marked, with the black windows showing the regions of the experimentally measured K-edges, and the red windows showing regions of the spectrum where collisional effects are the main contributor to the emission from a specific line. Figure 1: Experimental emission spectra. Experimentally measured K α intensities as a function of the spectrally resolved emission (horizontal axis) and X-ray pump photon energy (vertical axis) [23] , [24] . Emission from Al charge states 4 + to 8 + are marked, with the black windows showing the regions of the experimentally measured K-edges, and the red windows showing regions of the spectrum where collisional effects are the main contributor to the emission from a specific line. Full size image Simulations As the experimental results are collected over the duration of the X-ray pulse, which also heats and ionizes the sample, the analysis remains reliant on the accurate modelling of the evolution of the plasma system under the intense X-ray irradiation. Therefore, we simulate the experiment using the SCFLY collisional-radiative code [8] , [9] , which has proved capable of modelling the non-local thermodynamic equilibrium evolution of X-ray FEL-irradiated samples [23] , [24] , [25] , [26] , [27] . The basic parameters of the simulation have been reported previously [23] , [24] , [25] . The X-ray pulse is modelled via a Gaussian time distribution with a full-width at half-maximum pulse length of 80 fs. The simulations of the K α peaks away from resonance are seen to not depend on the specific time structure of the pulse, and varying the pulse length down to 60 fs, or the shape to that of a square pulse yields identical results to those reported, provided the total energy contained in the pulse is left unchanged. The time structure of the evolution of the system is simulated over a period of 200 fs in 50 time steps, and the total spectrum is obtained by integrating the emission from all steps. In the experiment, the sample was irradiated over a range of different intensities determined by the spatial focusing profile of the X-ray beam. This distribution on target of the X-ray intensity was measured experimentally and is used to construct a two-dimensional (2D) intensity map of the surface of the emitting region of the sample [28] , [29] . In the calculations, the total emitting region is simulated by binning the target in 30 intensity bins, spanning over five orders of magnitude in intensity, each of which constitutes an independent atomic kinetics simulation. The spectra from these individual simulations are then weighted by the volume of the region irradiated at that intensity, and added together to simulate the emission observed experimentally on the detector. Such simulated emission spectra, pumped at photon energies of 1,590 and 1,630 eV, are shown as a function of time in Fig. 2 . Here the peak of the X-ray pump is set to t =0 (negative times are earlier). The comparison between the time-integrated calculated spectrum and the experimental measurement is given at the top of Fig. 2 , and illustrates an excellent agreement between the two, provided the higher collision rates are used in the calculation, as will be discussed shortly. We note that, while the FEL pump and the simple X-ray photoabsorption interaction channel enable us to accurately simulate the plasma evolution, the emission spectrum remains that of a sample, which is both inhomogeneously spatially heated, and which is also evolving in time. 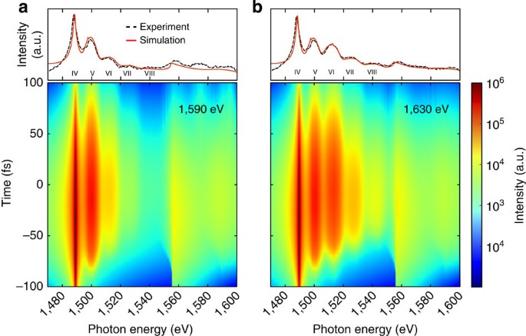Figure 2: Simulated emission spectra. The three-dimensional (3D) simulated spectrum from the target sample, shown both resolved in time and time-integrated, is in excellent agreement with the experimental measurement, provided the higher collision rates are used (see text andFig. 3). The Gaussian FEL pulse has a full-width at half-maximum of 80 fs and its peak is placed att=0. Ina, the system is shown to be pumped at 1,590 eV, for which lines IV and V can be pumped directly, while lines VI and above emit because of collisional processes. Inb, the system is pumped at 1,630 eV and lines VII and above emit because of collisional ionization. The relatively weak feature just below 1,560 eV is Kβemission. Figure 2: Simulated emission spectra. The three-dimensional (3D) simulated spectrum from the target sample, shown both resolved in time and time-integrated, is in excellent agreement with the experimental measurement, provided the higher collision rates are used (see text and Fig. 3 ). The Gaussian FEL pulse has a full-width at half-maximum of 80 fs and its peak is placed at t =0. In a , the system is shown to be pumped at 1,590 eV, for which lines IV and V can be pumped directly, while lines VI and above emit because of collisional processes. In b , the system is pumped at 1,630 eV and lines VII and above emit because of collisional ionization. The relatively weak feature just below 1,560 eV is K β emission. Full size image The opacity of the emitting region is modelled via the escape factor formalism, with a line-of-sight target thickness of 1 μm. The escape factor formalism was shown to be an adequate way to model the opacity in these conditions, provided the X-ray pumping occurs above the cold Al K-edge (1,550 eV); more detailed radiation transfer calculations are in turn required to model the K-L resonance transitions [27] . The bandwidth of the X-ray pulse is 0.4%, determined experimentally [23] . The calculations presented use the modified version of the Ecker–Kröll model (mEK) [30] for the IPD, which has been previously observed to be the most accurate model for both describing the evolution of the physical system, as well as for reproducing the observed spectra [25] . The collision rates used are those in ref. 5 . Collisional ionization The experiment is sensitive to collisional processes. To show this, let us consider the emission line VI, photo-pumped at an X-ray photon energy of 1,590 eV. The atomic configuration that produces emission line VI is K 1 L 6 . In the experiment, K-shell vacancies can only be created via photoionization, since the temperature of the system heated by the LCLS is never sufficient for the thermal ionization of the K-shell of Al to be significant. Given that the K-edge of configuration K 2 L 6 is at 1,610 eV (see Fig. 1 ), the configuration K 1 L 6 cannot be created via photoionization from this ground state with X-ray photons at 1,590 eV. Hence, one might expect to observe no emission from line VI while the X-ray pump remains below 1,610 eV. As we see from Fig. 2a , however, a non-negligible amount of emission from line VI is produced at this pump wavelength. In contrast, the emission from line V is determined by the photoionization of configuration K 2 L 7 , which has a K-edge at 1,575 eV, and is energetically allowed. This results in a significant production of ions in the K 1 L 7 configuration, which in turn gives rise to the strong emission from line V. We now note that, although the electron temperature is insufficient for K-shell ionization, it is large enough for significant L-shell collisional ionization to take place. This provides an alternative channel for the creation of the line VI emitting configuration K 1 L 6 from the photoionization of K 2 L 7 , rather than from the energetically forbidden K 2 L 6 , via a two-step process: Clearly, this channel opens once the first step (photoionization) is possible, so that the intensity of emission line VI depends not only on the K-edge of charge state 5 + ( K 2 L 6 ) but also on the K-edge of the lower charge state 4 + ( K 2 L 7 ). Since multiple L-shell collisions can occur, albeit with decreasing probability, the intensity of a specific emission line will generally depend on the K-edge of all lower charge states. The ionic configuration K 1 L 7 is short-lived, with a lifetime determined primarily by the Auger recombination into K 2 L 5 , which takes place within about 2 fs. The amount of K 1 L 6 created in these conditions via the process described in equation (1) is then given through the competition between collisional and Auger processes, both of which compete to destroy state K 1 L 7 . Importantly, this means that, provided the emission intensities are a good map of the charge state populations they correspond to, and provided we can neglect higher-order collisional effects, the ratio of neighbouring emission lines pumped at an X-ray photon energy that lies between the K-edges of the two states can yield directly the ratio between the collisional ionization rate and the rate of Auger decay for a specific charge state. Since the Auger rates are an atomic property of the ion, such a measurement provides a straightforward method to extract collision rates in a dense, strongly coupled plasma. We plot in Fig. 3 the intensity of the emission lines IV through VIII as a function of the pump X-ray photon energy. The emission is normalized to the the main K α line and is offset for clarity. While each of these charge states has an observable K-edge determined by the minimum photon energy necessary to photoionize a 1 s electron in an Al ion of given atomic configuration, we further observe that higher charge states display multiple such edges, that is, thresholds for the emission intensity at photon energies well below that of the K-edge. These higher-order edges appear at the photon energies of the K-edges of lower charge states, and are driven by collisional ionization of the L-shell electrons, via the chain process described in equation (1). For example, the experimental emission from line VII clearly shows three distinct thresholds at the K-edge energies of charge states 4 + , 5 + and 6 + . 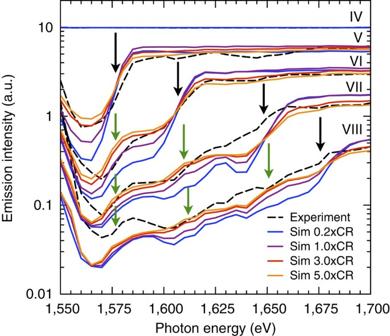Figure 3: Charge-state-resolved emission intensity. Emission intensity of lines IV–VIII as a function of FEL pump photon energy. The line intensities are normalized to the first Kαline, and are displaced for clarity. Superimposed on the experimental emission intensities are the simulations conducted with the SCFLY code, using a range of scaling factors for the collisional ionization rates of 0.2, 1, 3 and 5. Black arrows indicate the position of the experimental K-edge of the line-generating charge state, while green arrows indicate the position of the K-edges of all lower charge states. Figure 3: Charge-state-resolved emission intensity. Emission intensity of lines IV–VIII as a function of FEL pump photon energy. The line intensities are normalized to the first K α line, and are displaced for clarity. Superimposed on the experimental emission intensities are the simulations conducted with the SCFLY code, using a range of scaling factors for the collisional ionization rates of 0.2, 1, 3 and 5. Black arrows indicate the position of the experimental K-edge of the line-generating charge state, while green arrows indicate the position of the K-edges of all lower charge states. Full size image Ionization potential depression An accurate modelling of the evolution of the system, as well as that of collisional ionization processes, requires the positions of the K-edges to be calculated correctly a range of charge states and plasma conditions. This is because the K-edges need to be known for the spectroscopic model here described to be applicable, but more importantly, because the IPD determines the energy required to ionize bound electrons, and also affects the collision rates via determining the free-electron temperature and density distribution. As previously reported in ref. 25 the mEK IPD model, which we also employ here, is capable of reproducing the measured experimental K-edges with good accuracy. More precisely, we see from Fig. 3 that for lines IV and V the IPD is overestimated by at most a few eV (position of edge in simulations is lower than that of the experiment), while for lines VI and above the IPD is underestimated by at most 5–10 eV. We note that other commonly used IPD models, such as that of Stewart and Pyatt [31] or based on the ion-sphere model [32] , tend to significantly underestimate the IPD, and can misplace the position of the K-edge by as much as 50 eV for charge state 7 + (ref. 25 ). Recently, several theoretical calculations of the IPD applicable to the experimental conditions shown here were conducted, the results of which are in better agreement with the trend of both the mEK model and the experimental edges as depicted in Fig. 3 (refs 33 , 34 , 35 ). The effect of collisional ionization can best be observed from the step-like features of the emission intensity of the various emission lines, as shown in Fig. 3 . In particular, the ratio between intensities of neighbouring lines near absorption edges is overwhelmingly dominated by collisional ionization within the time window of Auger decay. A higher emission intensity above the K-edge of a certain charge state in the calculations compared with the experiment is, therefore, indicative of too few collisions taking place (insufficient depopulation of the photo-pumped charge state), while for the below-edge case the same is true if the simulations yield a lower emission intensity than in the experiment (insufficient collisional population of a charge state that cannot be photo-pumped directly). An interesting consequence of this is that observing the emission above and below the absorption edge of a single line can be sufficient to estimate the rate of collisions taking place, and, in particular, whether or not this process is accurately reproduced by the theoretical models used in collisional-radiative calculations. This effect is clearly shown by the different calculations presented in Fig. 3 . We deduce from Fig. 3 that the standard model for collisional ionization yields rates that are consistently too small to explain the observed spectral emission for all the emission lines investigated (V–VIII). To evaluate the amount by which this process is underestimated, we have performed calculations for a range of scaled collision rates, where all the collisional ionization rates, as well as their inverse processes (or, equivalently, cross-sections) are multiplied by a factor of 0.2, 1, 3 or 5. All other parameters in the simulations are held constant. The results are shown by the various simulation lines in Fig. 3 , from which we see that the collision rates are underestimated by as much as a factor of 3 or more over the range of conditions investigated. We note that the changes in the collisional rates have no influence on the positions of the Al K-edges. Despite the spectrum being emitted from a plasma, which is inhomogeneously heated, both spatially and in time, we find that the individual lines that emit because of the collisional ionization of an Al ion with a K-shell hole do so in surprisingly well-defined plasma conditions. The reason for this lies in the high collisionality of the system, which is very quickly driven towards LTE. To see this, we plot in Fig. 4a the distribution of emission from the various intensities from within the focal spot, which contribute to the total emission from line VI when the sample is pumped at 1,590 eV, a process described in detail in the previous section. Unsurprisingly, low intensities from the fringes of the focal spot contribute little to the emission of the line, as an insufficient number of ions in the emitting charge states are created. Similarly, the highest intensities reached at the focus are also seen to contribute negligibly. Here copious amounts of the right charge states can be created; however, the fraction of the sample that interacts with the peak of the X-ray pulse is also very small, so that this emission is strongly overshadowed by the emission at intermediate intensities, which are representative of a much larger portion of the emitting plasma. This is why the intensity weighting distribution, shown in Fig. 4 , is seen to be peaked at intermediate intensities. For each value of the intensity we plot the free-electron temperature and density of the plasma in the conditions of peak emission of the line of interest during the pulse. While the various X-ray intensities heat regions of the sample to very different final temperatures and ionizations, we observe that the peak of the emission tends to always occur in very similar conditions, irrespective of the intensity. Hence, the parts of the sample that interact with high X-ray intensities will emit collisional lines VI (VII), shown in Fig. 4a,b , at earlier times, while those at low intensities will emit later, towards the end of the pulse. By weighting the electron temperatures and densities over all intensities via this distribution, we can extract the range of conditions in which the line was emitted across the whole plasma, that is, where the predominant amount of collisional ionization took place. For an X-ray pump photon energy of 1,590 eV, we find T =(27±4) eV, n e =(2.5±0.2) × 10 23 cm −3 for line VI. Similarly, the emission from line VII, when the plasma is pumped at 1,630 eV (driven by the collisional process K 1 L 6 +collision→ K 1 L 5 + e − ), occurs at T =(35±4) eV and n e =(2.9±0.2) × 10 23 cm −3 . 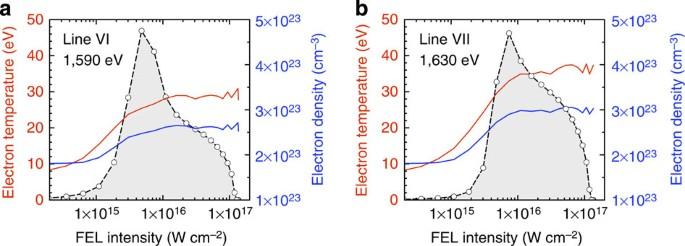Figure 4: Sample conditions during peak emission. Conditions in the sample at which emission occurs from charge states that are generated predominantly via the collisional ionization of L-shell electrons, inafor line VI at a pump photon energy of 1,590 eV, and inbfor line VII at a pump of 1,630 eV. Despite the integrated nature of the experiment, the majority of the line emission occurs at very well-defined electron temperatures and densities. Figure 4: Sample conditions during peak emission. Conditions in the sample at which emission occurs from charge states that are generated predominantly via the collisional ionization of L-shell electrons, in a for line VI at a pump photon energy of 1,590 eV, and in b for line VII at a pump of 1,630 eV. Despite the integrated nature of the experiment, the majority of the line emission occurs at very well-defined electron temperatures and densities. Full size image Our collisional-radiative calculations assume instant thermalization of the Auger and photoelectrons to provide the instantaneous free-electron temperature and density. In reality, however, although they thermalize quickly, the Auger electrons, and to a much lesser extent the photoelectrons, will be nonthermal for a short period of time, during which their effect on the collisional ionization process will be different to that of the thermal free electrons. A large relative population of energetic Auger electrons could then skew the interpretation of the experimental results, provided their collisional cross-section was significantly different to that of the cooler, thermal electrons, because collisional ionization from the Auger electrons is not included separately in our calculations. To estimate the size of this effect, we have separated the Augers from the thermal electrons in the simulation and thus relaxed the assumption of instant thermalization, so that now, in order to thermalize, an Auger electron must either collisionally ionize an ion in the system or collide with the thermal electrons. This ionization is tracked alongside that of the thermal electrons and is plotted in Fig. 5 as a function of time during the FEL pulse, at a photon energy of 1,630 eV. Importantly, we find that the population of each charge state peaks at a time when the collisional ionization due to the thermal electrons is over an order of magnitude larger than that due to the Auger electrons. Hence, we conclude that the instant thermalization assumption is overall valid in these conditions, and that the error introduced in the evaluation of the collision rates is not significant. 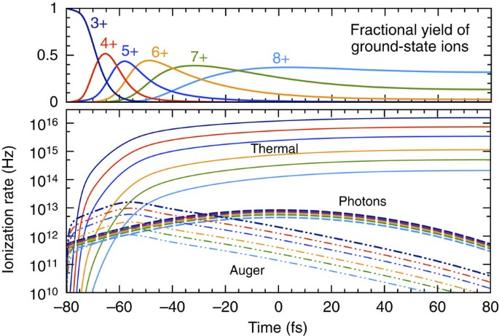Figure 5: Calculated ionization rates. Comparison between collisional ionization rates of Auger and thermal electrons during the FEL pulse for charge states 3+to 8+, at a photon energy of 1,630 eV. Each charge state population is seen to peak at times when thermal ionization exceeds the ionization driven by the Auger electrons by over an order of magnitude. Figure 5: Calculated ionization rates. Comparison between collisional ionization rates of Auger and thermal electrons during the FEL pulse for charge states 3 + to 8 + , at a photon energy of 1,630 eV. Each charge state population is seen to peak at times when thermal ionization exceeds the ionization driven by the Auger electrons by over an order of magnitude. Full size image Recently, more advanced calculations of relaxation dynamics of the free-electron distribution in an FEL-driven system using a Fokker–Planck approach were reported in ref. 36 . At the highest densities at which they performed their calculations, of 10 22 atoms cm −3 , the authors report a persistent presence of nonthermal Auger and photoelectrons during the entire duration of the pulse. However, because of the high density of the system the populations of these high-energy electrons were seen to be very small compared with that of the thermal electron distribution, for all but the very beginning of the pulse. This observation is consistent with our simpler calculations. Moreover, our results are for solid-density Al, which has a six-times higher atomic density, for which thermalization times should be even shorter. Perhaps surprisingly, the effect of nonthermal electrons in the distribution was also seen to initially lower the observed rates of impact ionization [36] . The reason for this is that in the instant thermalization approximation, all the absorbed energies that do not go into ionization contribute directly to the temperature, whereas for nonthermal distributions some of that energy is syphoned off to the high-energy electrons, leading to a cooler thermal electron component. Hence, were these effects significant, one would expect to overestimate the experimental collisional ionization rates in the calculation rather than underestimate them, as is the case of the results reported here. In conclusion, we have described a spectroscopic method to extract femtosecond collisional ionization rates in dense plasmas using the unique characteristics of an X-ray FEL, namely its high intensity, narrow bandwidth and wavelength tunability. By comparing emission intensities of lines produced from neighbouring charge states, one of which is photo-pumped above its K-edge, the other below, the collisional ionization rate can be clocked to the Auger decay rate of a core hole, providing, in principle, a plasma-model-independent reference window for the collisional event. Recent experimental emission measurements on solid-density Al plasmas at LCLS show that the emission from charge states pumped below their respective K-edge is systematically underestimated by our collisional-radiative calculations in the regions where the measurements are sensitive to collisional effects. In the present measurements, opacity effects prevent us from extracting the collisional rate directly from the emission spectrum; therefore, we have conducted a full non-local thermodynamic equilibrium spectral calculation, including opacity via the escape factor formalism. We observe that the measurement is consistent with a too small collisional ionization rate used in the modelling, and are able to match the experimental results extremely well, with the exception of small discrepancies in the modelling of the IPD on the order of 5–10 eV, provided we assume the collisional ionization rates are larger by a factor between three and five. While nonthermal collisional effects, primarily driven by energetic Auger electrons, are an important contributing factor to the collisionality of the system at early times in the plasma evolution, our current calculations indicate that their effect should be small compared with the much larger thermal electron distribution at the times when most of the relevant emission intensities are produced. Regardless, we wish to stress that more detailed investigations, aimed at better quantifying the effect of nonthermal electron distributions on transition rates on ultrashort timescales, are certainly necessary in the context of studying collisional dynamics on X-ray FELs. Finally, we calculate that the plasma conditions in which the spectrum is sensitive to collisional effects has very well-defined electron temperatures and densities, despite the time- and space-integrated nature of the experiment. This is primarily because of the strong collisionality driving the system rapidly towards LTE, so that charge state populations, and hence peak emissions, are closely linked to the plasma temperature. Hence, this technique affords, for the first time, the possibility to measure charge-state-specific collisional ionization rates in well-defined conditions in dense, strongly coupled plasmas. How to cite this article: Vinko, S. M. et al . Investigation of femtosecond collisional ionization rates in a solid-density aluminium plasma. Nat. Commun. 6:6397 doi: 10.1038/ncomms7397 (2015).